Structural transformation and catalytic hydrogenation activity of amidinate-protected copper hydride clusters Copper hydrides are important hydrogenation catalysts, but their poor stability hinders the practical applications. Ligand engineering is an effective strategy to tackle this issue. An amidinate ligand, N,N′-Di(5-trifluoromethyl-2-pyridyl)formamidinate (Tf-dpf) with four N-donors has been applied as a protecting agent in the synthesis of stable copper hydride clusters: Cu 11 H 3 (Tf-dpf) 6 (OAc) 2 ( Cu 11 ) with three interfacial μ 5 -H and [Cu 12 H 3 (Tf-dpf) 6 (OAc) 2 ]·OAc ( Cu 12 ) with three interstitial μ 6 -H. A solvent-triggered reversible interconversion between Cu 11 and Cu 12 has been observed thanks to the flexibility of Tf-dpf. Cu 11 shows high activity in the reduction of 4-nitrophenol to 4-aminophenol, while Cu 12 displays very low activity. Deuteration experiments prove that the type of hydride is the key in dictating the catalytic activity, for the interfacial μ 5 -H species in Cu 11 are involved in the catalytic cycle whereas the interstitial μ 6 -H species in Cu 12 are not. This work highlights the role of hydrides with regard to catalytic hydrogenation activity. Copper hydrides have historically been studied for their exciting structural chemistry and applications in hydrogenation catalysis and hydrogen-storage technology [1] , [2] , [3] , [4] , [5] , [6] , [7] . Recently, intense attention has been paid to synthesize atomically precise copper hydride clusters. A series of copper hydride clusters with bidentate ligands have been reported, which contain bridging ( μ -H), capping ( μ 3 -H) and interstitial ( μ (4−6) -H) hydrides [8] , [9] , [10] , [11] , [12] , [13] , [14] , [15] , [16] . The precise control over number of hydrides and their arrangements within these copper hydride clusters could provide valuable possibilities in modulating their catalytic hydrogenation activity. However, these copper hydride clusters are usually not stable enough and lose their identity quickly in solution [17] , [18] , [19] , which presented synthetic difficulties and limited their wide application. Surface organic ligands are critical in the construction and stabilization of atomically precise metal nanoclusters [20] , [21] , [22] , [23] , [24] , [25] , [26] , [27] , ligand engineering is an important approach in promoting the stability of copper hydrides. Envisioning multidentate amine ligands could provide stronger protection to metal clusters due to their multiple binding sites and their anionic nature which is helpful for ligating cationic metal ions [28] , [29] , [30] , [31] , [32] , we chose an amidinate ligand, N,N′-Di(5-trifluoromethyl-2-pyridyl)formamidinate (Tf-dpf) containing four N-donors, as the protecting agent for copper hydride clusters. Such a strong protection of ligand shell favors the high stability of copper hydride clusters. Moreover, Tf-dpf has a flexible linear structure favoring the generation of metal cluster diversity [30] , which may be constructive in establishing structure-property relationships in terms of hydrogenation catalysis. Herein, we report two amidinate-protected copper hydride clusters Cu 11 H 3 (Tf-dpf) 6 (OAc) 2 ( Cu 11 ) and [Cu 12 H 3 (Tf-dpf) 6 (OAc) 2 ]·OAc ( Cu 12 ), and their reversible interconversion (Fig. 1 ). The hydride positions in Cu 11 and Cu 12 were further confirmed by a machine-learning model based on convolutional neural networks (CNN) and trained on published structures of copper hydride clusters from neutron diffraction. It is quite unexpected that Cu 11 showed high activity in the reduction of 4-nitrophenol (4-NP) to 4-aminophenol (4-AP), while Cu 12 displayed very low activity. Structural determination of these two clusters revealed that the type of hydride is the key in dictating the catalytic activity. Cu 11 has three interfacial μ 5 -H and Cu 12 has three interstitial μ 6 -H. Deuterated catalytic experiments confirmed that the μ 5 -H of Cu 11 is involved in the catalytic cycle whereas the μ 6 -H of Cu 12 is not active . These findings are not only helpful for understanding the catalytic mechanism, but also instructive for the design and synthesis of efficient hydrogenation catalysts. Fig. 1: The structure of Tf-dpf ligand and the solvent-induced interconversion of Cu 11 and Cu 12 . The chemical structure of Tf-dpf ( a ) and the structural transformation between Cu 11 and Cu 12 ( b ). Color legend of b : light blue, Cu; red, Hydride; white, Tf-dpf ligand. Full size image Synthesis and characterization HTf-dpf ligand was synthesized by heating the mixture of 5-(trifluoromethyl)-2-aminopyridine and excess triethyl orthoformate (TEOF) at 120 °C under nitrogen atmosphere (Supplementary Fig. 1 ) [33] . The preparation of Cu 12 involves the direct reduction of a mixture of Cu(OAc) and HTf-dpf/Et 3 N with a mild reducing agent, Ph 2 SiH 2 in a mixed CH 2 Cl 2 /CH 3 OH solvent. Cu 11 was obtained by changing the reaction solvent to CH 2 Cl 2 /DMSO (dimethylsulfoxide), and then crystallized from CH 2 Cl 2 and n-hexane. 1 H NMR spectroscopic analysis of Cu 11 (Supplementary Fig. 2a ) and Cu 12 (Supplementary Fig. 3a ) in CD 3 OD identified four sets of aromatic resonances corresponding to Tf-dpf ligands. Three OAc − in Cu 12 are divided into two groups in a 2:1 ratio based on their environments. Three hydrides in Cu 11 gave 1 H NMR signals at 2.34 (2H) and 3.15 (1H) ppm, and similar 1 H NMR shifts were found at 1.46–2.80 ppm for [Cu 20 H 11 (S 2 P(OiPr) 2 ) 9 ] [17] , and 2.18-3.44 ppm for [Cu 29 Cl 4 H 22 (Ph 2 phen) 12 ]Cl (Ph 2 phen = 4, 7-diphenyl-1,10-phenanthroline) [34] . The observed values of Cu 12 at 5.64 (2H) and 7.16 (1H) ppm are comparable to those in Cu 28 H 16 (dppe) 4 ((4-isopropyl)thiophenol) 4 (CH 3 CO 2 ) 6 Cl 2 at 3.4-6.3 ppm [35] , and the encapsulated hydrides in [Cu 8 H{S 2 CC(CN) 2 } 6 ] 5− and [Cu 8 H{S 2 C(NEt 2 )} 6 ] − at 7.02 and 7.6 ppm [36] , [37] , respectively. In addition, 19 F NMR of Cu 11 (Supplementary Fig. 2b ) and Cu 12 (Supplementary Fig. 3b ) in CD 3 OD show one singlet at −63.28 and −63.88 ppm, respectively (free HTf-dpf presents at −60.21 ppm, Supplementary Fig. 1b ), suggesting that the six Tf-dpf ligands in Cu 11 and Cu 12 are in similar environments, respectively. As shown in Fig. 2a , the positive ESI-MS spectrum of Cu 11 shows two prominent peaks, corresponding to the molecular ion [Cu 11 H 3 (Tf-dpf) 6 (OAc) 2 ] + ( m / z = 2819.64) and [Cu 11 H 3 (Tf-dpf) 5 (OAc) 2 ] + ( m / z = 2484.56). The spectrum of Cu 12 gave signal of molecular ion [Cu 12 H 3 (Tf-dpf) 6 (OAc) 2 ] + at m / z = 2882.51 (Fig. 2b ). The observed isotopic patterns of the clusters are in perfect agreement with the simulated. UV–vis absorption spectra of Cu 11 and Cu 12 in MeOH display three prominent absorption bands at 238, 288, and 340 nm, which are corresponding to the intraligand transitions of the Tf-dpf ligand, as similar bands are found in HTf-dpf (Supplementary Fig. 4 ). Fig. 2: ESI-MS of Cu 11 and Cu 12 in MeOH. Mass spectra of Cu 11 ( a ) and Cu 12 ( b ), inset: the measured (black trace) and simulated (red trace) isotopic distribution patterns of the corresponding the molecular ion peaks. Full size image To our surprise, Cu 11 and Cu 12 are very stable under ambient conditions. In the solid state, they are air and moisture stable (Supplementary Fig. 5 ). In addition, Cu 11 and Cu 12 are stable in solution (even in polar solvents such as CH 2 Cl 2 ) for 2 weeks (Supplementary Fig. 6 ). 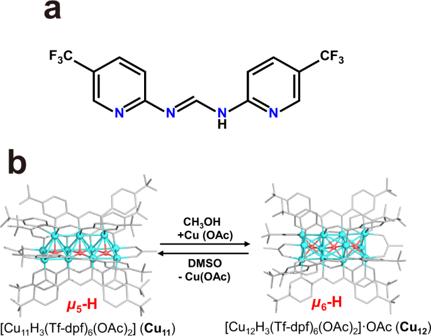Fig. 1: The structure of Tf-dpf ligand and the solvent-induced interconversion of Cu11and Cu12. The chemical structure of Tf-dpf (a) and the structural transformation betweenCu11andCu12(b). Color legend ofb: light blue, Cu; red, Hydride; white, Tf-dpf ligand. Molecular structures Single-crystal X-ray diffraction (SCXRD) structural analysis (Supplementary Table 1 ) revealed that Cu 11 comprises a Cu 11 H 3 (Tf-dpf) 6 (OAc) 2 cluster (Fig. 3a and Supplementary Fig. 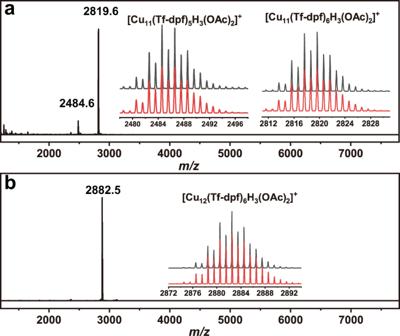Fig. 2: ESI-MS of Cu11and Cu12in MeOH. Mass spectra ofCu11(a) andCu12(b), inset: the measured (black trace) and simulated (red trace) isotopic distribution patterns of the corresponding the molecular ion peaks. 7 ), wherein six Tf-dpf ligands are ligated to Cu 11 ( μ 5 -H) 3 core in a linear pattern (four in motif A and two in motif B) with Cu–N bond lengths ranging from 2.026(4) to 2.131(4) Å (Supplementary Table 2 ). Two OAc − anions bind the two copper atoms at the ends of the linear Cu 11 ( μ 5 -H) 3 unit, giving the Cu−O bond lengths of 2.021(4) to 2.038(4) Å. The metal core of Cu 11 could be regarded as the fusion of three edge-sharing rectangular pyramids. The Cu…Cu distances of the Cu 11 skeleton range from 2.428(1) to 2.749(1) Å. Fig. 3: Molecular structures of Cu 11 and Cu 12 . Total structure of Cu 11 H 3 (Tf-dpf) 6 (OAc) 2 ( a ) and [Cu 12 H 3 (Tf-dpf) 6 (OAc) 2 ] + ( b ). Schematic representation of the binding modes of Tf-dpf in Cu 11 and Cu 12 ( c ). Color legend: light blue, Cu; green, F; blue, N; pink, O; gray, C; red, Hydride. Full size image The structure of Cu 12 includes a [Cu 12 H 3 (Tf-dpf) 6 (OAc) 2 ] + cationic cluster (Fig. 3b ) and a OAc − counter anion (Supplementary Fig. 8 ). The coordination modes of OAc − in Cu 12 are similar to that of Cu 11 , with the Cu–O bond lengths ranging from 2.111(5) to 2.120(4) Å. The six Tf-dpf ligands in Cu 12 adopt distorted motif A binding mode, with the Cu–N bond ranging from 2.000(5)–2.096(5) Å. The metal core of Cu 12 could be regarded as the fusion of three face-sharing octahedra. Moreover, the 12 copper atoms in Cu 12 are typical hexagonal close-packed type structure with ABAB packing mode (Supplementary Fig. 9 ). Cu…Cu distances of Cu 12 skeleton range from 2.497(1)–2.764(1) Å, which is much longer than that of Cu 11 . Shorter Cu…Cu contact in Cu 11 could be attributed to the linear coordination mode of Tf-dpf, while Tf-dpf adopts zigzag coordination mode in Cu 12 to form relatively longer Cu…Cu contacts (average 2.657 Å) as shown in Fig. 3c . These Cu…Cu distances observed in Cu 12 is comparable to the average Cu…Cu contact of 2.66 Å in the Cu 6 octahedral structures [38] . Neural network prediction of hydride sites Even though the location of H atoms by SCXRD is difficult, the hydrides in Cu 11 and Cu 12 could be estimated based on the charge distribution in their cluster frameworks and refined freely. Although attempts to grow single crystals suitable for neutron diffraction were unsuccessful, we applied a recently developed machine-learning model based on CNN to confirm the hydride location. The CNN method can quickly predict hydride occupancy in a Cu cluster given the heavy-atom coordinates [39] , [40] . We fed the SCXRD-determined positions of heavy-atoms into the CNN model and predicted the most probable sites in the two clusters. As shown in Fig. 4 , the CNN model predicted close-to-1 occupancies in three sites for both the Cu 11 and Cu 12 clusters. The locations of these top three sites are shown in Fig. 4 insets; indeed, they exactly match the sites determined from SCXRD. Further density functional theory (DFT) geometry optimizations confirmed the stability of these clusters, as the cluster framework was well maintained after structural relaxation with hydrides at the predicted sites, and the SCXRD and DFT structures were in good agreement (Supplementary Table 2 ). For the sites with probability around 0.7–0.9, we would normally consider them as well, but the Cu 11 and Cu 12 clusters are much smaller and their structures are much simpler, quite resembling the structures in our training set. So the most probable three sites from our machine-learning model happen to be the most viable model that agrees with the SCXRD and is further confirmed by DFT. Fig. 4: Neural network prediction of hydride sites. Probability distribution of hydride occupancy in the possible sites as predicted by convolutional neural network: a Cu 11 H 3 ; b Cu 12 H 3 . Insets show the probabilities of the top-ranked sites and their positions in the clusters before DFT optimization. Color legend: Cu, dark salmon; Hydride, white. Full size image In Cu 11 , three hydrides are disposed in the center of Cu 4 square with an approximate square pyramidal μ 5 coordination mode. Of note, the positions of the three μ 5 -H in Cu 11 relative to the centers of Cu 4 squares differ slightly: the middle one is right in the center of Cu 4 square and the other two are deviated from the centers of Cu 4 squares (close to the OAc − ). The Cu-H distances were found in the range from 1.61(6) to 2.02(7) Å. In Cu 12 , three hydrides are disposed in the center of Cu 6 octahedra with a μ 6 -H coordination mode. Similar to that in Cu 11 , the middle H was found to be right in the center of Cu 6 octahedron, while the other two show offsets closing to the OAc − . The Cu- μ 6 -H distance in Cu 12 ranges from 1.71(8) to 2.02(6) Å. Interconversion Interestingly, it was found that the interconversion between Cu 11 and Cu 12 could be triggered by solvents. The interconversion involves the adding a Cu + ion to Cu 11 or leaving of a Cu + ion from Cu 12 . Dissolving Cu 12 in DMSO led to the leaving of a Cu + ion to form Cu 11 , while the reaction of Cu 11 with CuOAc (1 equiv) in CH 3 OH converted it back to Cu 12 . The interconversion was not affected by O 2 for the same interconversion was observed both in the air and under nitrogen atmosphere. The flexible arrangement of the N donors of Tf-dpf makes such an interconversion possible, which allows keeping stable ligation to metal ions in adjusting to the structural changes between Cu 11 and Cu 12 . To better understand the cluster-to-cluster transformation process, we monitored the cluster core transformation process ( Cu 12 to Cu 11 ) by ESI-MS measurements (Fig. 5a ). The MeOH solution of Cu 12 features one prominent peak attributed to [Cu 12 H 3 (Tf-dpf) 6 (OAc) 2 ] + . The freshly prepared Cu 12 solution in DMSO showed peaks corresponding to [Cu 11 H 3 (Tf-dpf) 6 (OAc) 2 ] + along with a weak peak attributed to [Cu 11 H 3 (Tf-dpf) 5 (OAc) 2 ] + within 5 min. Then the peaks of Cu 11 keep increasing with time, and after 120 min the spectrum features only prominent peaks of Cu 11 while the peak of Cu 12 disappeared, indicating the complete conversion from Cu 12 to Cu 11 . Fig. 5: Conversion of Cu 12 to Cu 11 . a Changes in the ESI-MS spectrum of Cu 12 in DMSO. b Changes in the 19 F NMR spectrum of Cu 12 in DMSO- d 6 . Full size image We then monitored a solution of Cu 12 in DMSO- d 6 at room temperature by measuring its 19 F NMR spectra at different times. A slight upfield shift of ∼ 2.6 ppm of Cu 12 and Cu 11 was found in DMSO- d 6 compared with in CD 3 OD. As shown in Fig. 5b , the signal at −61.24 ppm of Cu 12 gradually disappeared, while that at −60.68 ppm of Cu 11 gradually grew with increasing time, indicating a transformation of Cu 12 to Cu 11 in DMSO at room temperature. Based on the integration ratios relative to the internal standard, the conversion of Cu 12 to Cu 11 is virtually quantitative. Given the different numbers of Cu atoms in Cu 11 and Cu 12 , the transformation between the two clusters is not isomerization. As shown in (Supplementary Fig. 10 ), the OAc − only binds two out of the three terminal copper atoms of the Cu 12 core, and the other one copper atom could be regarded as an unsaturated site. Thus, it is hypothesized that the transformation of Cu 12 to Cu 11 is attributed to the binding ability of DMSO, which anchors on the unsaturated copper atom and removes it from the cluster. As a result, the binding mode of Tf-dpf in Cu 12 is distorted motif A, which leads to the twisting of two Cu 3 units and then the framework rearrangement to form Cu 11 (Fig. 6 ). Moreover, the conversion of Cu 11 to Cu 12 through adding CuOAc in CH 3 OH proves that Cu 11 is likely to combine free Cu ions to generate Cu 12 (Supplementary Fig. 11 ). Fig. 6: Hypothetic step-by-step transformation from Cu 12 to Cu 11 . a , b DMSO takes away an unsaturated copper atom; b , c two Cu 3 units of Cu 12 twist for 60° along with the binding mode of Tf-dpf changes; c , d the translation of linear Cu 3 unit. Color legend: light blue, red, and green Cu; gray, Tf-dpf; black, Hydride. Full size image Hydrogenation catalysis Synthesis of anilines or amines from the corresponding nitro compounds is an important process in both of the laboratory and the chemical industry due to their versatility in several biologically active natural products, pharmaceuticals, and dyes [41] . Transition metal-catalyzed hydrogenation is an important route for the transformation of nitro groups to amine groups [42] , [43] . Thus, the reduction of 4-NP to 4-AP by NaBH 4 was chosen as a model reaction to investigate the catalytic performance of Cu 11 and Cu 12 . Considering that Cu 11 and Cu 12 are insoluble in water, this catalytic reaction belongs to heterogeneous catalysis. The reduction process monitored by measuring the intensity change of 400 nm peak (4-NP) in UV/vis absorption spectroscopy. As the catalytic reaction proceeded in the presence of Cu 11 , the intensity of 400 nm peak decreased rapidly and disappeared within 10 min (Fig. 7a ), indicating the complete conversion of 4-NP to 4-AP ( λ max = 295 nm in water). In comparison, only 5% 4-NP could be reduced to 4-AP with equivalent Cu 12 catalyst even when the time was extended to 30 min, and the completion of reduction of 4-NP to 4-AP needed 10 h (Supplementary Fig. 12 ). It is quite interesting that two copper hydride clusters with similar structures show distinctly different activity in the hydrogenation reaction (Fig. 7b ), which prompts us to pay efforts in mechanism study in terms of the role of hydrides. Fig. 7: Catalytic performance of Cu 11 and Cu 12 . a UV–Vis spectra showing gradual reduction of 4-NP catalyzed by Cu 11 . b Plot of −ln(c/c 0 ) vs. reaction time during the reduction of 4-NP with Cu 11 and Cu 12 catalysts. c ESI-MS of Cu 12 after catalysis with NaBD 4 . Inset: the comparison of the measured (black trace) and simulated isotopic distribution patterns of [Cu 12 H 3 (Tf-dpf) 6 Cl 2 ] + (green, 2834.5), [Cu 12 H 3 (Tf-dpf) 6 (OAc)Cl] + (blue, 2858.5), and [Cu 12 H 3 (Tf-dpf) 6 (OAc) 2 ] + (red, 2882.5). d ESI-MS of Cu 11 after catalysis with NaBD 4 . Inset: the comparison of the measured (black trace) and simulated (red trace) isotopic distribution patterns of [Cu 11 HD 2 (Tf-dpf) 5 (OAc) 2 + Na] + (2844.6) and [Cu 11 HD 2 (Tf-dpf) 5 (OAc)] + (2762.6). Full size image Three major steps were generally thought to be involved in transition metal-catalyzed reduction of 4-NP to 4-AP [41] , [44] , and the formation of [M]–H species as well as the B–H bond cleavage was considered to be the rate-determining step. Therefore, we carried out an experiment using Cu 11 and Cu 12 as the catalysts for the reduction of 4-NP to 4-AP with NaBD 4 in place of NaBH 4 . In the cases of Cu 12 , no peak belongs to deuterated cluster was found in the ESI-MS spectrum after catalysis with NaBD 4 (Fig. 7c ), which indicates that the encapsulated μ 6 -H of Cu 12 were shielded from interaction with substrates. Therefore, Cu 12 showed very low catalytic activity. On the contrary, the ESI-MS of Cu 11 after catalysis with NaBD 4 showed new peaks at 2762.6 and 2844.6 in addition to the expected peak of 2484.6 ([Cu 11 H 3 (Tf-dpf) 5 (OAc) 2 ] + ) (Fig. 7d ). These two new peaks could be attributed to [Cu 11 HD 2 (Tf-dpf) 6 (OAc)] + and [Cu 11 HD 2 (Tf-dpf) 6 (OAc) 2 + Na] + , respectively, which indicates that hydrides in Cu 11 were replaced by D atoms from NaBD 4 , i.e., the μ 5 -H species of Cu 11 were involved in the catalytic cycle. These facts reveal that the high catalytic activity of Cu 11 is related to the formation of μ 5 -H species on the cluster. Moreover, it is noted that Cu 11 is relatively robust and can be re-used after centrifugation. 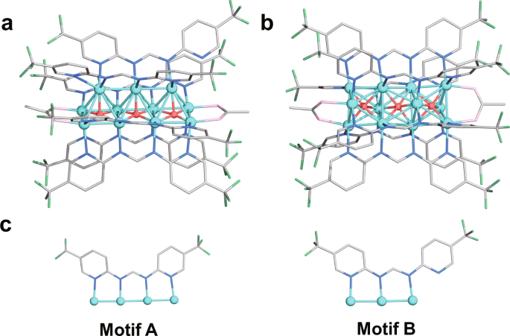Fig. 3: Molecular structures of Cu11and Cu12. Total structure of Cu11H3(Tf-dpf)6(OAc)2(a) and [Cu12H3(Tf-dpf)6(OAc)2]+(b). Schematic representation of the binding modes of Tf-dpf inCu11andCu12(c). Color legend: light blue, Cu; green, F; blue, N; pink, O; gray, C; red, Hydride. Even after seven cycles, Cu 11 retains its high activity (Supplementary Table 3 ). Previously reported copper hydride clusters including Stryker’s reagent are usually moisture- and air-sensitive. Other copper hydride clusters such as [Cu 3 H(dppm) 3 (OAc) 2 ] [45] , [46] and [Cu 8 H 6 (dppy) 6 ](OTf) 2 [7] are stable in solution for less than 3 days. Cu 11 and Cu 12 are stable in CH 2 Cl 2 for at least 2 weeks, their good stability makes them promising copper hydride catalysts for various applications. Overall, Cu 11 and Cu 12 present a pair of valuable copper hydride clusters for correlating the structures and properties. They have identical amidinate ligands, similar metal atom arrangement, but different hydride location and distinct catalytic performance, which demonstrates the importance of the location of hydrides for efficient hydrogenation catalysis [45] . This information will be instructive in the design, synthesis and selection high performance hydrogenation catalysts. In summary, we have synthesized two stable copper hydride clusters Cu 11 and Cu 12 with the flexible amidinate ligand Tf-dpf. Because the multidentate amine ligand Tf-dpf has a negative charge and four binding N donors, it could provide strong binding to metal centers. Such a strong protection of ligand shell favors the high stability of copper hydride clusters. The compositions of these two title clusters have only one copper atom difference, but their structures and hydride positions are different. Cu 11 and Cu 12 show totally distinct catalytic performance in the reduction of 4-NP to 4-AP. Cu 11 bearing μ 5 -H is very active while Cu 12 with μ 6 -H display very low activity. Deuterated catalytic experiments prove that the hydrides at different location play key a role in the catalytic cycles. This work presents valuable information for understanding the hydrogenation process of copper hydride catalysts at atomic level, which helps optimize the design and synthesis of stable and active copper hydride catalysts. Chemicals and materials 5-(trifluoromethyl)-2-aminopyridine (97%) was purchased from Meryer. Triethyl orthoformate (TEOF, 99%) and Et 3 N (99%) were purchased from Aladdin. H 2 SiPh 2 was purchased from Bidepharm, China. CuOAc (93%) was purchased from TCI. Other reagents employed were purchased from Sinopharm Chemical Reagent Co. Ltd. (Shanghai, China). All chemical reagents employed were used without further purification. Synthesis of N,N′-Di(5-trifluoromethyl-2-pyridyl)formamidine (HTf-dpf) Excess TEOF (1.8571 g, 17.5 mmol) was added to of 5-(trifluoromethyl)-2-aminopyridine (3.2422 g, 20.0 mmol) and heated at 120 °C under a low nitrogen stream for 5 h. The excessed TEOF and ethanol formed during the reaction were distilled off, and the product was recrystallized from petroleum ether/methanol (5:1). Yield: 2.97 g, 89%. Anal. UV–Vis ( λ , nm): 231; 267; 323. 1 H NMR (400 MHz, DMSO- d 6 , δ , ppm): 11.41 (s, 1H, –CH–), 9.77 (s, 1H, NH), 8.70 (s, 2H, py), 8.11–8.08 (dd, 2H, py), 7.22 (s, 2H, py). 19 F NMR (400 MHz, DMSO- d 6 , δ , ppm): −60.21. 13 C NMR (400 MHz, DMSO- d 6 , δ , ppm): 151.70, 146.17, 136.20, 128.70, 126.00, 123.31, 120.61. Synthesis of [Cu 12 (Tf-dpf) 6 (OAc) 2 H 3 ]·OAc (Cu 12 ) In total, 3 ml CH 2 Cl 2 /CH 3 OH (v:v = 2:1) mixture of Cu(OAc) (24 mg, 0.2 mmol), HTf-dpf (0.1 mmol, 33.4 mg), and excess Et 3 N (20 ul) was stirred for 5 min first, then H 2 SiPh 2 (0.1 mmol, 18 ul) was added. The solution color changed from green to yellow in 10 min. 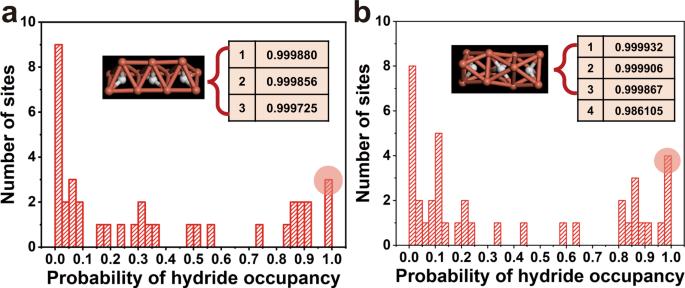Fig. 4: Neural network prediction of hydride sites. Probability distribution of hydride occupancy in the possible sites as predicted by convolutional neural network:aCu11H3;bCu12H3. Insets show the probabilities of the top-ranked sites and their positions in the clusters before DFT optimization. Color legend: Cu, dark salmon; Hydride, white. The mixture was stirred for 3 h and evaporated to dryness to give a yellow solid, which was washed with n-hexane (3 × 2 ml), then dissolved in 4 ml CH 2 Cl 2 /CH 3 OH (v:v = 3:1). The resulted solution was centrifuged for 2 min at 9000 r/min, and the yellow supernatant was collected and subjected to diffusion with n-hexane to afford light yellow crystals after 2 days in 27.4 mg, 56% yield (based on Cu). Anal. UV–Vis ( λ , nm): 238; 288; 341. ESI-MS (CH 3 OH): 2882.51 ([Cu 12 (Tf-dpf) 6 (OAc) 2 H 3 ] + ). 1 H NMR (400 MHz, CD 3 OD, δ , ppm): 8.95 (m, 6H, –CH–), 8.55 (m, 12H, py), 7.59–7.57 (m, 12H, py), 7.23–7.20 (m, 12H, py), 7.16 (s, 1H, hydride), 5.64 (s, 2H, hydride), 3.59 (s, 3H, –CH 3 ), 2.68 (s, 6H, –CH 3 ). 19 F NMR (400 MHz, CD 3 OD, δ , ppm): −63.88. Synthesis of Cu 11 (Tf-dpf) 6 (OAc) 2 H 3 (Cu 11 ) In total, 3 ml CH 2 Cl 2 /DMSO (v:v = 5:1) mixture of Cu(OAc) (24 mg, 0.2 mmol), HTf-dpf (0.1 mmol, 33.4 mg), and excess Et 3 N (20 ul) was stirred for 5 min first, then H 2 SiPh 2 (0.1 mmol, 18 ul) was added. The solution color changed from green to yellow in 10 min. The mixture was stirred for 3 h and evaporated to remove the CH 2 Cl 2 solvent. 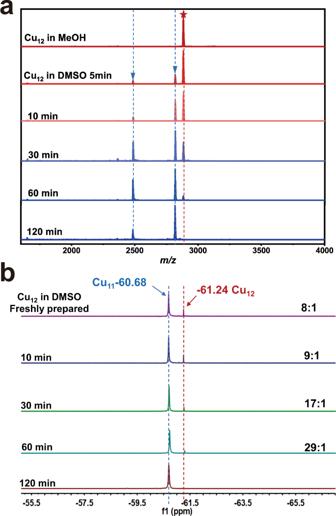Fig. 5: Conversion of Cu12to Cu11. aChanges in the ESI-MS spectrum ofCu12in DMSO.bChanges in the19F NMR spectrum ofCu12in DMSO-d6. The crude product was washed by 5 ml CH 2 Cl 2 /n-hexane (v:v = 1:4) for three times, then dissolved in 4 ml CH 2 Cl 2 . The resulted solution was centrifuged for 2 min at 9000 r/min, and the orange supernatant was collected and subjected to diffusion with n-hexane to afford light orange crystals after 2 days in 24.2 mg, 47% yield (based on Cu). Anal. UV–Vis ( λ , nm): 240; 287; 338. ESI-MS (CH 3 OH): 2819.64 ([Cu 11 (Tf–dpf) 6 (OAc) 2 H 3 ] + ) and 2484.56 ([Cu 11 (Tf-dpf) 5 (OAc) 2 H 3 ] + ). 1 H NMR (400 MHz, CD 3 OD, δ , ppm): 8.98–8.54 (m, 12H, –CH– and py), 7.59–7.50 (m, 12H, py), 7.21–7.17 (m, 12H, py), 3.15 (s, 1H, hydride), 2.60 (s, 6H, –CH 3 ), 2.34 (s, 2H, hydride). 19 F NMR (400 MHz, CD 3 OD, δ , ppm): −63.28. Catalytic reduction of 4-nitrophenol The water solution of 4-NP (1 ml, 20 mM), Cu 11 or Cu 12 (1 mg) was mixed, and the mixture was stirred for 10 min at room temperature. Time-resolved UV–vis spectra were taken immediately after the addition of NaBH 4 solid (50 mg, 1.3 mmol). The progress of the reaction was tracked by monitoring the change in intensity of 4-NP peak at 400 nm as a function of time. After reaction of Cu 11 , the reaction solution was centrifuged, and the catalysts was washed with 3 ml H 2 O for three times. Then the catalysts solid was dried under reduced pressure and re-used as fresh. Neural network prediction of hydride sites We employed the recently developed deep-learning model to predict hydride sites in our clusters. The model was based on CNN and trained on Cu-H clusters with hydride sites determined by neutron diffraction. This model takes as input the heavy-atom coordinates of a cluster from the single-crystal X-ray diffraction and then outputs the occupancy for each possible hydride site in the cluster. The training data are based on 23 different copper hydride clusters from the Cambridge Structural Database whose hydride locations have been determined by neutron diffraction. The 23 structures were further chunked into 674 boxes of possible hydride sites that were used for training of CNN. The details of the CNN and its architecture can be found in the previous work [39] , [40] and their Supporting Information. The trained CNN can classify a possible site for hydride in a given cluster with accuracy higher than 94%. In the present work, the X-ray structures of the Cu 11 and Cu 12 clusters (namely, coordinates of Cu, C, N, F, and O in the cluster) were used as input into the machine-learning model which then predicted hydride occupancies and ranked the hydride sites. Since there are only three hydrides in the Cu 11 and Cu 12 clusters, one can simply pick the top-ranked sites and examine the top three by inspection, followed by DFT geometry optimization for confirmation using the VASP code. Physical measurements UV–Vis absorption spectra was recorded on cary5000. Mass spectra were recorded on a high-resolution Fourier transform ICR spectrometer with an electrospray ionization source in positive mode. Nuclear magnetic resonance data were recorded on a Bruker Avance II spectrometer (500 MHz). X-ray crystallography Intensity data of compounds Cu 11 and Cu 12 were collected on an Agilent SuperNova Dual system (Cu Kα) at 173 K. Absorption corrections were applied by using the program CrysAlis (multi-scan). The structures of Cu 11 and Cu 12 were solved by direct methods. Non-hydrogen atoms except solvent molecules and counteranions were refined anisotropically by least-squares on F 2 using the SHELXTL program. For Cu 12 , the -CF 3 groups (F7–F9, F22–F24) were disordered over two sites with an occupancy factor of 0.5/0.5. SQUEEZE routine in PLATON was employed in the structural refinements due to large solvent voids. In addition, isor and rigu constraints have been applied due to geometric requirements of the ligands. 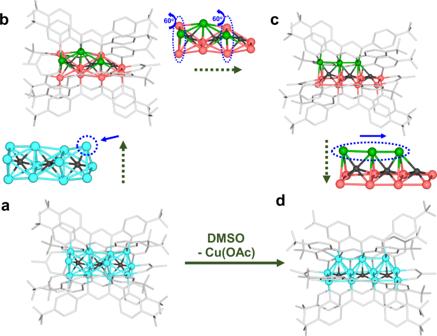Fig. 6: Hypothetic step-by-step transformation from Cu12to Cu11. a,bDMSO takes away an unsaturated copper atom;b,ctwo Cu3units ofCu12twist for 60° along with the binding mode of Tf-dpf changes;c,dthe translation of linear Cu3unit. Color legend: light blue, red, and green Cu; gray, Tf-dpf; black, Hydride. 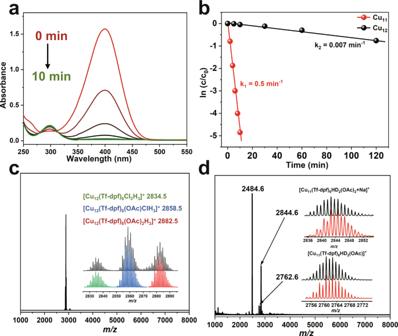Fig. 7: Catalytic performance of Cu11and Cu12. aUV–Vis spectra showing gradual reduction of 4-NP catalyzed byCu11.bPlot of −ln(c/c0) vs. reaction time during the reduction of 4-NP withCu11andCu12catalysts.cESI-MS ofCu12after catalysis with NaBD4. Inset: the comparison of the measured (black trace) and simulated isotopic distribution patterns of [Cu12H3(Tf-dpf)6Cl2]+(green, 2834.5), [Cu12H3(Tf-dpf)6(OAc)Cl]+(blue, 2858.5), and [Cu12H3(Tf-dpf)6(OAc)2]+(red, 2882.5).dESI-MS ofCu11after catalysis with NaBD4. Inset: the comparison of the measured (black trace) and simulated (red trace) isotopic distribution patterns of [Cu11HD2(Tf-dpf)5(OAc)2+ Na]+(2844.6) and [Cu11HD2(Tf-dpf)5(OAc)]+(2762.6). Computational methods DFT calculations were performed with the quantum chemistry program Turbomole V7.1 [47] . The Def2-SV(P) basis sets [48] were used for C, N, O, H, F. The Def2-TZVP basis sets [49] were used for Cu. Geometry optimization was done with the functional of Perdew, Burke and Ernzerhof [50] .